Functional and molecular interactions between ERK and CHK2 in diffuse large B-cell lymphoma Distinct oncogenic signalling cascades have been associated with non-Hodgkin lymphoma. ERK1/2 signalling elicits both transcriptional and post-transcriptional effects through phosphorylation of numerous substrates. Here we report a novel molecular relationship between ERK1/2 and CHK2, a protein kinase that is a key mediator of the DNA damage checkpoint that responds to DNA double-strand breaks. Our studies are the first to demonstrate the co-localization and overexpression of ERK1 /2 and CHK2 in diffuse large B-cell lymphoma (DLBCL). The physical interaction between ERK and CHK2 was highly dependent on phosphorylated Thr 68 of CHK2. Concurrent administration of an ERK inhibitor enhances the antitumour activity of CHK2 inhibition in both a human DLBCL xenograft model as well as primary human DLBCL cells. Our data suggest a functional interaction between ERK and CHK2 and support the potential combined therapeutic targeting of ERK and CHK2 in human DLBCL. Recent evidence implicates DNA repair and the genome integrity checkpoints as major barriers whose deregulation is largely responsible for the enhanced genetic instability of cancer cells [1] . The CHK2 kinase is a key mediator of the DNA damage checkpoint that responds to DNA double-strand breaks (DSBs). DNA DSBs induce the activation of ATM (ataxia telangiectasia mutated), which subsequently phosphorylates CHK2 on threonine 68 (ref. 2 ). Phosphorylation of CHK2 induces CHK2 dimerization, which is required for CHK2 activity. Once dimerized, CHK2 is further activated by autophosphorylation in trans at residues 383, 387, 546 and 516 (ref. 2 ). CHK2 phosphorylates a range of proteins involved in cell cycle control and apoptosis including cdc25A, cdc25C, Mdmx, p53, BRCA1, PML, E2F1, and phosphatase 2A (ref. 2 ). CHK2 also mediates stabilization of the FoxM1 transcription factor to stimulate expression of DNA repair genes [3] . Cells derived from CHK2-deficient mice exhibit defects in their ability to delay entry into S phase, sustain a G2 cell cycle arrest, and undergo apoptosis in response to DNA damage [4] . It is newly reported that CHK2, independent of p53 and DNA damage, is required for proper progression of mitosis, and for the maintenance of chromosomal stability in human somatic cells [5] . CHK2 can also protect genome integrity by promoting apoptosis through interacting with a number of other substrates. Inhibition of CHK2 by transfection of a dominant-negative CHK2 mutant or a chemical inhibitor, debromohymenialdesine, stabilizes centrosomes, maintains high cyclin B1 levels, and allows for a prolonged activation of Cdk1 (ref. 6 ). Under these conditions, multinuclear HeLa syncytia do not arrest at the G2/M boundary and rather enter mitosis and subsequently die during the metaphase of the cell cycle [6] . Therefore, inhibition of CHK2 can sensitize proliferating cells to chemotherapy-induced apoptosis. The first indication of the role of CHK2 in cancer came from a study that reported the presence of germline mutations in CHK2 in families with Li-Fraumeni Syndrome [7] . It has been subsequently shown that defects of CHK2 occur in subsets of diverse sporadic malignancies and predispose to several types of hereditary carcinomas [8] . However, there is increasing evidence that CHK2 is a cancer susceptibility gene, but not a tumour suppressor gene in the classical sense [9] , [10] . CHK2 is aberrantly and constitutively activated in invasive urinary bladder carcinomas, and the putative proapoptotic checkpoint signalling can be disabled by inactivation of CHK2 and/or p53 tumour suppressors in subsets of these tumours [8] . More than 50% of CHK2 was phosphorylated at Thr68 in surgically resected lung and breast tumour specimens from otherwise untreated patients [11] . Targeting of CHK2 with small interfering RNA prevents survivin release from the mitochondria and enhanced apoptosis following induction of DNA damage by ionizing radiation (IR) or doxorubicin and inhibits the growth of resistant in vivo tumours. Expression of a dominant negative CHK2 potentiates cytotoxicity in HCT116 colon carcinoma cells to doxorubicin [9] . These findings suggested that activated CHK2 manifests both tumour-suppressor functions as well as the capacity to promote tumour and cell survival [9] , [12] . Relatively little is known about the contribution of CHK2 or the efficacy of CHK2 inhibitor in diffuse large B-cell lymphoma (DLBCL). The extracellular signal-regulated kinases 1 and 2 (ERK1/2) regulate cell proliferation and survival. Deregulation of ERK signalling is associated with genomic instability and cancer [13] . In earlier work, we showed that ERK inhibition induced the apoptosis of human DLBCL cells and has marked antitumour activity in human DLBCL xenograft models, implying the potential role of targeting ERK in the therapy of DLBCL [14] . It was shown that disruption of ERK1/2 activation by pharmacologic MEK1/2 inhibitors results in a dramatic increase in apoptosis of hematopoietic malignant cells [15] , [16] . Considering that there is little data on CHK2 and ERK signalling in lymphoid malignancies, in this study, we explored the molecular mechanisms underlying the functional interaction between ERK2 and CHK2. Furthermore, we investigated the potential therapeutic efficacy of combining ERK and CHK2 inhibitors in a pre-clinical model of DLBCL. We report here that the interaction between ERK and CHK2 was highly dependent on phosphorylated Thr 68 of CHK2 and that concurrent administration of an ERK inhibitor enhances the antitumour activity of CHK2 inhibition in human DLBCL. ERK1/2 and CHK2 are highly expressed in human DLBCL To examine the expression of both ERK1/2 and CHK2 in human DLBCL, we performed immunohistochemistry analysis to evaluate the ERK1/2 and CHK2 protein levels on 50 primary DLBCL specimens and 24 reactive lymph nodes. The expression of ERK1/2 and CHK2 was examined in the adjacent slides from the same sample. The DLBCL was further classified into germinal centre B-cell (GCB) and activated B-cell (ABC) subtypes, according to well-accepted immunohistochemistry-based algorithms [17] , [18] . Based on the criteria defined in the Methods, the specimens were divided into three staining groups: negative, low and high. 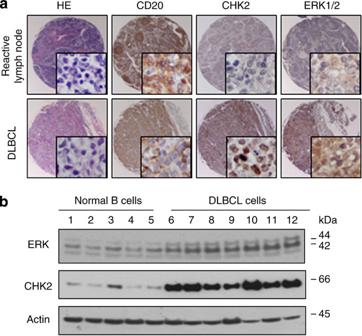Figure 1: ERK1/2 and CHK2 protein levels are elevated in human DLBCLs. (a) Representative fields of reactive germinal centre B-cell centroblasts and DLBCL tissue arrays immunohistochemically stained with anti-CD20, anti-CHK2 and anti-ERK1/2 antibodies as indicated. Low (original magnification, X20) and high (original magnification, X400) power views of CD20, CHK2, and ERK1/2 expression in reactive germinal centre B-cell centroblasts and DLBCL cells (immunoperoxidase stains). H&E staining was used for morphologic examination. (b) The correlation between ERK1/2 and CHK2 expression was shown in normal B cells and DLBCL cells. Five cases of normal B cells from different donors and seven DLBCL cells were lysed and subjected to the western blot analysis with the indicated antibodies. 1–5, Normal B cells from different donors. 6, OCI-LY3; 7,SUDHL4; 8, SUDHL6; 9, Farage; 10, Pfeiffer; 11, Toledo; 12, Karpars-422. As summarized in Table 1 , ERK1/2 levels are markedly elevated in 98% of all the DLBCL and 100% of the GCB subtype DLBCL samples as compared with the normal GCB cells of the reactive lymph nodes (21%). CHK2 is also elevated in 100% of the GCB DLBCL samples as compared with the normal GCB cells of reactive lymph nodes (46%). Interestingly, our correlation analysis revealed that ERK1/2 expression levels in human DLBCL samples are strongly correlated with CHK2 protein levels (Pearson correlation coefficient ρ =0.737, P <0.0001). Representative sections of human DLBCL arrays are shown in Figure 1a . These data indicate that increased coexpression of ERK1/2 and CHK2 may be associated with the development of DLBCL. These data were further confirmed by western blot analysis in normal B cells and DLBCL cells ( Fig. 1b ). Together, ERK1/2 and CHK2 protein levels appear to be elevated in the vast majority of DLBCL, supporting their value as potential therapeutic targets. Table 1 Immunohistological analysis of ERK1/2 and CHK2 expression in DLBCL and normal GCB cells. Full size table Figure 1: ERK1/2 and CHK2 protein levels are elevated in human DLBCLs. ( a ) Representative fields of reactive germinal centre B-cell centroblasts and DLBCL tissue arrays immunohistochemically stained with anti-CD20, anti-CHK2 and anti-ERK1/2 antibodies as indicated. Low (original magnification, X20) and high (original magnification, X400) power views of CD20, CHK2, and ERK1/2 expression in reactive germinal centre B-cell centroblasts and DLBCL cells (immunoperoxidase stains). H&E staining was used for morphologic examination. ( b ) The correlation between ERK1/2 and CHK2 expression was shown in normal B cells and DLBCL cells. Five cases of normal B cells from different donors and seven DLBCL cells were lysed and subjected to the western blot analysis with the indicated antibodies. 1–5, Normal B cells from different donors. 6, OCI-LY3; 7,SUDHL4; 8, SUDHL6; 9, Farage; 10, Pfeiffer; 11, Toledo; 12, Karpars-422. Full size image Inhibition of ERK and CHK2 increases DLBCL cells apoptosis It has been reported that inhibition of CHK2 expression attenuated DNA damage-induced cell cycle checkpoints and enhanced apoptotic activity in HEK293 cells [10] , [19] . We asked whether inhibition of CHK2 would induce apoptosis in DLBCL cells. The CHK2 Inhibitor II shows 1,000-fold greater selectivity for the CHK2 serine/threonine kinase than for the Cdk1/B and CK1 kinases and was first discovered to be a potent, selective small molecule showing radioprotection towards human T cells [20] . CHK1 and CHK2 are structurally unrelated yet functionally belong to the checkpoint kinase family [1] . Therefore, we compared CHK1 phosphorylation with CHK2 phosphorylation after CHK2 Inhibitor II treatment. Phosphorylation of CHK2 at Thr68 by ATM functions as a surrogate marker for CHK2 activation [11] , [21] . We found that different doses of CHK2 inhibitor II specifically inhibit CHK2 phosphorylation at Thr68 at different time course, but not CHK1 phosphorylation ( Fig. 2a,b ). These data indicated that the CHK2 inhibitor II is specific for the inhibition of CHK2 activity. Exposure of SUDHL4, SUDHL6 and Farage cells to 5 μM CHK2 inhibitor II resulted in the apoptosis of less than 30% cells ( Fig. 2c ). We previously demonstrated that less than 30% DLBCL cells underwent apoptosis when exposed to 20 μM of a novel ERK inhibitor [14] . Because DLBCL has two major subtypes (ABC versus GC), we subsequently examined the efficacy of combining CHK2 inhibitor II with ERK inhibitor in both ABC (for example, OCI-LY3) and GC-type (Farage, SUDHL4 and SUDHL6) cells. Treatment with combination of CHK2 inhibitor II and ERK inhibitor resulted in substantially more apoptosis compared with treatment of either drug alone ( Fig. 2c ). Similar result was obtained in OCI-LY3 cells ( Supplementary Fig. S1 ). DNA DSBs are demonstrated by examining the phosphorylation of histone H2AX on Ser139 residues (designated γH2AX) [15] . Exposure to either the ERK inhibitor or CHK2 inhibitor II alone induced a modest increase in H2AX phosphorylation, whereas co-administration of both inhibitors dramatically increased H2AX phosphorylation. Apoptosis by the combination of these two inhibitors was also demonstrated by examining PARP cleavage ( Fig. 2d ). 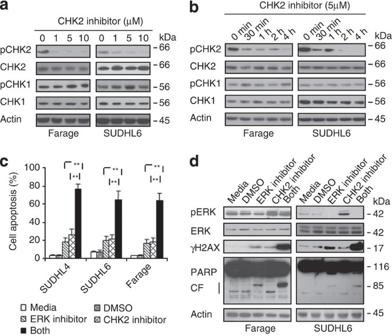Figure 2: Inhibition of ERK and CHK2 increases cell apoptosis. (a) The specificity of CHK2 inhibitor II. Farage and SUDHL6 cells were treated with different doses of CHK2 inhibitor II in RPMI 1640 complete medium for 4 h. The levels of pCHK1, CHK1, pCHK2 and CHK2 in the total cell lysates were monitored by immunoblotting with the indicated antibodies. (b) Farage and SUDHL6 cells were treated with 5 μM CHK2 inhibitor II in RPMI 1640 complete medium for different time course. The levels of pCHK1, CHK1, pCHK2 and CHK2 were examined by immunoblotting. (c) SUDHL4, SUDHL6 or Farage cells were exposed to 5 μM CHK2 inhibitor II or 20 μM ERK inhibitor alone or in combination for 72 h after which the percentage of apoptotic cells was determined by Annexin V analysis as described in Methods. Data show means and s.d. from at least three separate experiments.Pvalues were calculated using a paired Studentt-test. **Indicates values significantly greater (P<0.01) than treatment with either agent alone. (d) Farage or SUDHL6 cells were treated as described inc, after which whole cells were lysed and subjected to western blot analysis to monitor expression of γH2AX and cleavage of PARP. CF, cleavage fragments. Figure 2: Inhibition of ERK and CHK2 increases cell apoptosis. ( a ) The specificity of CHK2 inhibitor II. Farage and SUDHL6 cells were treated with different doses of CHK2 inhibitor II in RPMI 1640 complete medium for 4 h. The levels of pCHK1, CHK1, pCHK2 and CHK2 in the total cell lysates were monitored by immunoblotting with the indicated antibodies. ( b ) Farage and SUDHL6 cells were treated with 5 μM CHK2 inhibitor II in RPMI 1640 complete medium for different time course. The levels of pCHK1, CHK1, pCHK2 and CHK2 were examined by immunoblotting. ( c ) SUDHL4, SUDHL6 or Farage cells were exposed to 5 μM CHK2 inhibitor II or 20 μM ERK inhibitor alone or in combination for 72 h after which the percentage of apoptotic cells was determined by Annexin V analysis as described in Methods. Data show means and s.d. from at least three separate experiments. P values were calculated using a paired Student t -test. **Indicates values significantly greater ( P <0.01) than treatment with either agent alone. ( d ) Farage or SUDHL6 cells were treated as described in c , after which whole cells were lysed and subjected to western blot analysis to monitor expression of γH2AX and cleavage of PARP. CF, cleavage fragments. Full size image ERK and CHK2 physically interact with each other in DLBCLs To better understand the relationship between ERK and CHK2 in vivo , we conducted double-immunofluorescence analysis of ERK1/2 and CHK2 in human primary DLBCLs to detect their co-localization. 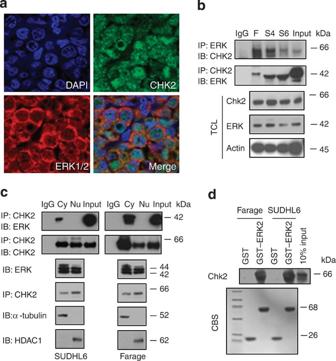Figure 3: ERK1/2 and CHK2 physically interact with each other. (a) Co-localization of ERK1/2 and CHK2 in human lymphoma tissues. Double immunofluorescent staining for CHK2 (green) and ERK (red) at X600 magnification indicates that there is strong overlapping in human lymphoma tissues. DAPI, 4′,6-diamidino-2-phenylindole; Merge, merged image of CHK2, ERK1/2, and DAPI. (b) ERK1/2 associates with CHK2 in cells. Farage, SUDHL4 and SUDHL6 cells were subjected to immunoprecipitation using either anti–ERK1/2 or anti-CHK2 antibody, followed by immunoblotting with indicated antibodies. TCL, total cell lysate. F, Farage; S4, SUDHL4; S6, SUDHL6. (c) Equal amounts of cytoplasmic (Cy) and nuclear fraction (Nu) were immunoprecipitated with anti-CHK2 antibody followed by immunoblotting with anti-ERK1/2 or anti-CHK2 antibody. Tubulin and HDAC1 were used as markers of the cytoplasmic and nuclear fractions respectively. (d) ERK2 associates with CHK2in vitro. GST-fused ERK2 was immobilized onto GlutathioneS-transferase beads and then incubated with Farage or SUDHL6 cell lysates. Immunoblotting was followed using anti-CHK2 antibody. As shown in Figure 3a , CHK2 was localized to both the cytoplasmic and nuclear factions of DLBCLs, and ERK was predominately localized in the cytoplasm of DLBCLs. In addition, endogenous ERK and CHK2 were predominately co-localized in the cytoplasm of human DLBCLs. We next examined whether ERK physically associated with CHK2. We were able to detect the reciprocal co-immunoprecipitation of endogenous ERK1/2 with CHK2 in Farage, SUDHL4 and SUDHL6 cells ( Fig. 3b ). Consistent with their co-localization, the endogenous ERK and CHK2 proteins co-immunoprecipitated predominately from the cytoplasm fraction of SUDHL6, Farage and OCI-LY3 cells ( Fig. 3c ; Supplementary Fig. S2a ). To further confirm this interaction and to demonstrate a direct physical interaction, in vitro glutathione S -transferase (GST) fusion protein pull-down assays were performed. We showed that the GST–ERK2 fusion protein was able to pull down CHK2 ( Fig. 3d ). Taken together, these data establish the physical interaction between ERK1/2 and CHK2. Figure 3: ERK1/2 and CHK2 physically interact with each other. ( a ) Co-localization of ERK1/2 and CHK2 in human lymphoma tissues. Double immunofluorescent staining for CHK2 (green) and ERK (red) at X600 magnification indicates that there is strong overlapping in human lymphoma tissues. DAPI, 4′,6-diamidino-2-phenylindole; Merge, merged image of CHK2, ERK1/2, and DAPI. ( b ) ERK1/2 associates with CHK2 in cells. Farage, SUDHL4 and SUDHL6 cells were subjected to immunoprecipitation using either anti–ERK1/2 or anti-CHK2 antibody, followed by immunoblotting with indicated antibodies. TCL, total cell lysate. F, Farage; S4, SUDHL4; S6, SUDHL6. ( c ) Equal amounts of cytoplasmic (Cy) and nuclear fraction (Nu) were immunoprecipitated with anti-CHK2 antibody followed by immunoblotting with anti-ERK1/2 or anti-CHK2 antibody. Tubulin and HDAC1 were used as markers of the cytoplasmic and nuclear fractions respectively. ( d ) ERK2 associates with CHK2 in vitro . GST-fused ERK2 was immobilized onto Glutathione S -transferase beads and then incubated with Farage or SUDHL6 cell lysates. Immunoblotting was followed using anti-CHK2 antibody. Full size image Thr 68 of CHK2 mediates the interaction between ERK and CHK2 Because CHK2 inhibitor II modestly induced the apoptosis of DLBCL cells, we asked whether CHK2 inhibition could affect the interaction between ERK and CHK2. Different doses of CHK2 inhibitor II dramatically diminished the physical interaction between ERK and CHK2 ( Fig. 4a ). Because the CHK2 inhibitor II specifically inhibits CHK2 phosphorylation at Thr68, this indicated that CHK2 phosphorylation at Thr68 is involved in the physical interaction between ERK and CHK2. We examined the CHK2 Thr68 to Ala (T68A) mutant that was established previously [22] . Due to high levels of CHK2 protein in DLBCL cells and the technical difficulty in transfecting SUDHL4 and SUDHL6 cells using liposomal or electroporation methods, we expressed CHK2 wild type (WT) and its mutant T68A in both HEK293 and HeLa cells. Wild-type CHK2 co-immunoprecipitated with ERK2, but the mutant CHK2 T68A did not ( Fig. 4b ). These results are further corroborated by GST pull-down experiments. 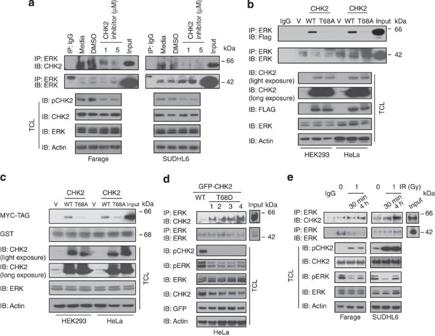Figure 4: CHK2 Thr68 is required for the physical interaction between ERK1/2 and CHK2. (a) Farage and SUDHL6 cells were treated with CHK2 inhibitor II in RPMI 1640 complete medium for 4 h. The cell lysates were subjected to immunoprecipitation with anti–ERK1/2 or anti-CHK2 antibody followed by immunoblotting with anti-CHK2 or anti-ERK1/2 antibody. The expression of pCHK2, CHK2 or ERK1/2 was monitored by immunoblotting of the total cell lysates. Actin was used as a loading control. (b) HEK 293 and HeLa cells were transiently transfected with the expression plasmids as indicated. At 24 h post-transfection, immunoprecipitation was performed using anti-ERK1/2 antibody followed by immunoblotting with anti-Flag or anti-ERK1/2 antibody. (c) HEK 293 and HeLa cells were transiently transfected with the Flag (MYC)-tagged CHK2 expression plasmids as indicated. At 24 h post-transfection, Cell lysates were incubated with GST–ERK2 bound to glutathione-Sepharose 4B beads at 4 °C for 1 h. The beads were washed intensively, and the bound proteins were detected by immunoblotting with an anti-Myc antibody. The GST fusion proteins were detected with anti-GST. (d) HeLa cells were transiently transfected with GFP–CHK2–WT or GFP–CHK2–T68D expression plasmids as indicated. At 24 h post-transfection, immunoprecipitation was performed using anti-ERK1/2 antibody followed by immunoblotting with anti-CHK2 or anti-ERK1/2 antibody. The expression of pCHK2,pERK1/2,CHK2, ERK1/2 or GFP was monitored by immunoblotting of the total cell lysates. Actin was used as a loading control. 1,2,3,4, four different clones. (e) Farage and SUDHL6 cells were treated or untreated with 1 Gy of IR) and collected 30 min or 4 h later for immunoprecipitation and western blotting analysis. Figure 4c shows that the GST–ERK2 protein can pull down CHK2 WT but not the T68A mutant. Mimicking T68 phosphorylation with a negatively charged amino-acid Asp (T68D) promoted ERK interaction with CHK2 ( Fig. 4d ). In addition, IR, which enhances CHK2 T68 phosphorylation, also increases their interaction ( Fig. 4e ). Together, these data demonstrated that Thr68 phosphorylation is required for the interaction between ERK and CHK2. Figure 4: CHK2 Thr68 is required for the physical interaction between ERK1/2 and CHK2. ( a ) Farage and SUDHL6 cells were treated with CHK2 inhibitor II in RPMI 1640 complete medium for 4 h. The cell lysates were subjected to immunoprecipitation with anti–ERK1/2 or anti-CHK2 antibody followed by immunoblotting with anti-CHK2 or anti-ERK1/2 antibody. The expression of pCHK2, CHK2 or ERK1/2 was monitored by immunoblotting of the total cell lysates. Actin was used as a loading control. ( b ) HEK 293 and HeLa cells were transiently transfected with the expression plasmids as indicated. At 24 h post-transfection, immunoprecipitation was performed using anti-ERK1/2 antibody followed by immunoblotting with anti-Flag or anti-ERK1/2 antibody. ( c ) HEK 293 and HeLa cells were transiently transfected with the Flag (MYC)-tagged CHK2 expression plasmids as indicated. At 24 h post-transfection, Cell lysates were incubated with GST–ERK2 bound to glutathione-Sepharose 4B beads at 4 °C for 1 h. The beads were washed intensively, and the bound proteins were detected by immunoblotting with an anti-Myc antibody. The GST fusion proteins were detected with anti-GST. ( d ) HeLa cells were transiently transfected with GFP–CHK2–WT or GFP–CHK2–T68D expression plasmids as indicated. At 24 h post-transfection, immunoprecipitation was performed using anti-ERK1/2 antibody followed by immunoblotting with anti-CHK2 or anti-ERK1/2 antibody. The expression of pCHK2,pERK1/2,CHK2, ERK1/2 or GFP was monitored by immunoblotting of the total cell lysates. Actin was used as a loading control. 1,2,3,4, four different clones. ( e ) Farage and SUDHL6 cells were treated or untreated with 1 Gy of IR) and collected 30 min or 4 h later for immunoprecipitation and western blotting analysis. Full size image CHK2 negatively regulates ERK activity The interaction of CHK2 and ERK suggests that they may regulate each other and ERK may be involved in CHK2-mediated DNA damage responses. This is also supported by our observation that ERK inhibitor potentiates CHK2 inhibitor-induced cell apoptosis. However, it is still unclear how these two proteins regulate each other and why co-treatment with ERK and CHK2 inhibitors increased cell apoptosis. To begin to address these questions, we next assessed whether inhibition of CHK2 regulates ERK. The CHK2 inhibitor II decreases CHK2 phosphorylation at Thr68 but increases ERK phosphorylation in SUDHL6, Farage and OCI-LY3cells ( Fig. 5a ; Supplementary Fig. S2b ). Furthermore, when CHK2 was genetically modified to inhibit Thr68 phosphorylation, a similar result was observed. 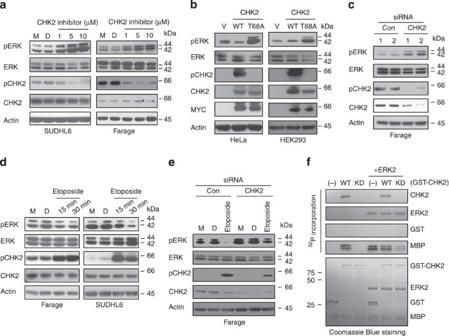Figure 5: Inhibition of CHK2 activity increases ERK1/2 phosphorylation. (a) SUDHL6 and Farage cells were treated with CHK2 inhibitor II in RPMI 1640 complete medium for 4 h. The levels of pCHK2, CHK2, pERK1/2 or ERK1/2 in the total cell lysates were monitored by immunoblotting with the indicated antibodies. (M, media; D, DMSO). (b) HeLa and HEK 293 cells were transiently transfected with the expression plasmids as indicated. At 24 h post-transfection, cell lysates were subjected to immunoblotting with anti-pERK1/2, anti-ERK1/2, anti-pCHK2, anti-CHK2 or anti-Myc antibody. (c) Knocking down of CHK2 increases ERK1/2 phosphorylation. Farage cells were transfected with control siRNA or CHK2 siRNA. At 72 h after transfection, the expression of pCHK2, CHK2, pERK1/2, ERK1/2, or Actin was monitored by immunoblotting. (d) Farage and SUDHL6 cells were treated with 5 μM Etoposide in RPMI 1640 complete medium for 15 or 30 min. Cell lysates were subjected to immunoblotting with anti-pERK1/2, anti-ERK1/2, anti-pCHK2 or anti-CHK2 antibody. (e) Knocking down of CHK2 attenuates the regulation of pERK by etoposide. Farage cells were transfected with control siRNA or CHK2 siRNA. At 48 h after transfection, Farage cells were treated with 5 μM Etoposide in RPMI 1640 complete medium for 30 min. Cell lysates were subjected to immunblotting with anti-pERK1/2, anti-ERK1/2, anti-pCHK2 or anti-CHK2 antibody. M, media; D, DMSO. (f) CHK2 directly inhibits ERK2-mediated phosphorylation through a kinase-independent mechanism. Purified wild-type (WT) or inactive (KD) GST–CHK2 and MBP were incubated in the absence or presence of ERK2, and protein phosphorylation was determined. Top panels: autoradiography of CHK2 and ERK2 autophosphorylation and phosphorylation of MBP. CHK2 does not inhibit ERK2 autophosphorylation but does inhibit ERK2-mediated phosphorylation of MBP. Bottom panels: Coomassie stain of CHK2, ERK2, and MBP in the kinase assays. GST was used as a control. Figure 5b showed that mutant T68A activated ERK but CHK2 WT failed to do so. In contrast, the phosphorylation-site mimic mutant T68D decreased ERK phosphorylation compared with CHK2 WT ( Fig. 4d ). These data indicated that ERK activity is regulated by CHK2 and the disruption of the physical interaction between ERK and CHK2 is necessary for the activation of ERK. Knockdown of CHK2 by its specific siRNA decreased CHK2 protein level and its phosphorylation; however, it also enhanced ERK phosphorylation ( Fig. 5c ). We next examined how ERK phosphorylation was affected when CHK2 phosphorylation was increased. It has been previously reported that etoposide is a potent activator of the DNA damage-signalling pathway [23] , [24] . Figure 5d shows that when CHK2 phosphorylation was increased after etoposide exposure, ERK phosphorylation was decreased. Knocking down of CHK2 attenuates the regulation of ERK by etoposide ( Fig. 5e ). In addition, while CHK2 phosphorylation at Thr68 was enhanced by IR, ERK phosphorylation was also decreased ( Fig. 4e ). Figure 5: Inhibition of CHK2 activity increases ERK1/2 phosphorylation. ( a ) SUDHL6 and Farage cells were treated with CHK2 inhibitor II in RPMI 1640 complete medium for 4 h. The levels of pCHK2, CHK2, pERK1/2 or ERK1/2 in the total cell lysates were monitored by immunoblotting with the indicated antibodies. (M, media; D, DMSO). ( b ) HeLa and HEK 293 cells were transiently transfected with the expression plasmids as indicated. At 24 h post-transfection, cell lysates were subjected to immunoblotting with anti-pERK1/2, anti-ERK1/2, anti-pCHK2, anti-CHK2 or anti-Myc antibody. ( c ) Knocking down of CHK2 increases ERK1/2 phosphorylation. Farage cells were transfected with control siRNA or CHK2 siRNA. At 72 h after transfection, the expression of pCHK2, CHK2, pERK1/2, ERK1/2, or Actin was monitored by immunoblotting. ( d ) Farage and SUDHL6 cells were treated with 5 μM Etoposide in RPMI 1640 complete medium for 15 or 30 min. Cell lysates were subjected to immunoblotting with anti-pERK1/2, anti-ERK1/2, anti-pCHK2 or anti-CHK2 antibody. ( e ) Knocking down of CHK2 attenuates the regulation of pERK by etoposide. Farage cells were transfected with control siRNA or CHK2 siRNA. At 48 h after transfection, Farage cells were treated with 5 μM Etoposide in RPMI 1640 complete medium for 30 min. Cell lysates were subjected to immunblotting with anti-pERK1/2, anti-ERK1/2, anti-pCHK2 or anti-CHK2 antibody. M, media; D, DMSO. ( f ) CHK2 directly inhibits ERK2-mediated phosphorylation through a kinase-independent mechanism. Purified wild-type (WT) or inactive (KD) GST–CHK2 and MBP were incubated in the absence or presence of ERK2, and protein phosphorylation was determined. Top panels: autoradiography of CHK2 and ERK2 autophosphorylation and phosphorylation of MBP. CHK2 does not inhibit ERK2 autophosphorylation but does inhibit ERK2-mediated phosphorylation of MBP. Bottom panels: Coomassie stain of CHK2, ERK2, and MBP in the kinase assays. GST was used as a control. Full size image We next investigated whether CHK2 directly inhibits ERK activity in vitro . GST–CHK2–KD is defective for kinase activity because of substitution of the catalytically essential Asp347 residue with Ala [25] . This mutation prevents autophosphorylation of CHK2 kinase activity [25] . In Figure 5f , in vitro kinase assays showed ERK2 and CHK2 WT can autophosphorylate and phosphorylate the generic kinase substrate, myelin basic protein (MBP). Interestingly, CHK2–KD was able to inhibit ERK2's ability to phosphorylate MBP but had no apparent effect on ERK2 autophosphorylation, indicating that ERK2 catalytic activity was intact. These findings indicate that CHK2 can directly inhibit ERK2's ability to phosphorylate downstream substrates by an activity-independent mechanism. Together, these findings establish that CHK2 negatively regulates ERK and suggest that inhibition of CHK2 is most effective in killing DLBCL cells if ERK functions are also inhibited. ERK inhibition enhances the activity of CHK2 inhibitors in vivo Next, we examined whether CHK2 inhibition cooperated with ERK inhibition in the treatment of DLBCL tumours in vivo . We established SUDHL6 DLBCL xenografts in 28 severe combined immunodeficient (SCID) mice (7 mice per group). Once the tumour reached the size of 60–163 mm 3 , we treated the mice every other day intraperitoneally with either vehicle, ERK inhibitor (5 mg kg −1 ), CHK2 inhibitor II (1 mg kg −1 ), or both ERK inhibitor and CHK2 inhibitor II for 20 days. At these doses, no lethal toxicity, significant weight loss or any gross abnormalities were observed among treated animals (data not shown). No evidence of tissue damage was detected by microscopic examination of mouse organs ( Supplementary Fig. S3 ). Both 5 mg kg −1 ERK inhibitor and 1 mg kg −1 CHK2 inhibitor II modestly inhibited tumour growth but combined treatment with ERK inhibitor and CHK2 inhibitor II resulted in a statistically significant suppression of tumour growth ( Fig. 6a,b ). Moreover, western blot analysis revealed that combined treatment with the ERK inhibitor and CHK2 inhibitors caused a striking increase in H2AX phosphorylation and PARP cleavage ( Fig. 6c ). This further confirmed that co-administration of the CHK2 inhibitor markedly potentiates DNA damage in DLBCL cells exposed to ERK inhibitor and this event precedes induction of extensive apoptosis. Immunohistochemical analysis of tumour sections showed that co-administration of the ERK and CHK2 inhibitors markedly reduced expression of the cell proliferation marker Ki67 whereas each inhibitor alone had slight impact ( Fig. 6d ). In addition, TdT-mediated dUTP nick end labelling (TUNEL) assay showed that the combined treatment with ERK inhibitor and CHK2 inhibitor II resulted in greater induction of apoptosis compared with either inhibitor alone ( Fig. 6d ). 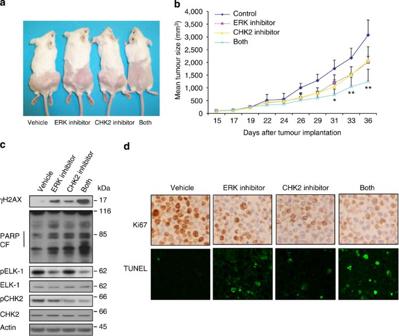Figure 6: Cotreatment with ERK inhibitor and CHK2 inhibitor II results in decreased tumour growth in a xenograft model. (a) 28 mice bearing s.c. tumours of SUDHL6 cells were divided into 4 groups (vehicle versus ERK inhibitor versus CHK2 inhibitor II versus combination), with 7 mice each. Representative mice were photographed before death to visually demonstrate tumour growth. (b) The average tumour volume of each group (n=7) with s.d. is shown as a function of time.Pvalues were calculated using a Studentt-test and statistical significance was determined when aPvalue less than 0.05 was attained. *P<0.05; **P<0.01 versus single treatments. (c) At the moment of mice death, xenograft tumours were excised, and the pooled protein extracts randomly from three mice of each group was subjected to western blot analysis using the indicated antibodies. (d) Tumour tissue sections were subjected to immunochemistry for Ki67 expression (original magnification, X400) and TUNEL staining (original magnification, X600). Figure 6: Cotreatment with ERK inhibitor and CHK2 inhibitor II results in decreased tumour growth in a xenograft model. ( a ) 28 mice bearing s.c. tumours of SUDHL6 cells were divided into 4 groups (vehicle versus ERK inhibitor versus CHK2 inhibitor II versus combination), with 7 mice each. Representative mice were photographed before death to visually demonstrate tumour growth. ( b ) The average tumour volume of each group ( n =7) with s.d. is shown as a function of time. P values were calculated using a Student t -test and statistical significance was determined when a P value less than 0.05 was attained. * P <0.05; ** P <0.01 versus single treatments. ( c ) At the moment of mice death, xenograft tumours were excised, and the pooled protein extracts randomly from three mice of each group was subjected to western blot analysis using the indicated antibodies. ( d ) Tumour tissue sections were subjected to immunochemistry for Ki67 expression (original magnification, X400) and TUNEL staining (original magnification, X600). Full size image Inhibition of ERK and CHK2 in human DLBCLs cells Because combined treatment of the CHK2 and ERK inhibitors is a candidate treatment strategy for human lymphomas, we wished to examine the effects of this combination on the apoptosis and viability of primary DLBCLs from human patients. Single cell suspensions were generated from two confirmed DLBCL lymph node biopsy specimens and exposed to either control (DMSO), ERK inhibitor, CHK2 inhibitor II or the combination of both inhibitors for 48 h. Co-treatment of the ERK and CHK2 inhibitors enhanced apoptosis of human primary DLBCL cells as compared with either inhibitor alone ( Fig. 7a ). Four cases of normal B cells are unresponsive to the inhibitor alone and the combination ( Supplementary Fig. S4a ). To further exclude the toxicity of the inhibitors in different cell phenotypes, immortalized untransformed fibroblasts (ID:GM04390, skin) were examined and insensitive to the combination of the inhibitors ( Supplementary Fig. S4b ). In addition, combined treatment with the ERK inhibitor and CHK2 inhibitor II dramatically reduced cells viability whereas the inhibitor administered individually had less effect ( Fig. 7b ). Therefore, these results are consistent with our DLBCL cell line and xenograft data and further support the concept that inhibition of ERK functions potentiates the antitumour activity of CHK2 inhibition in human DLBCLs. 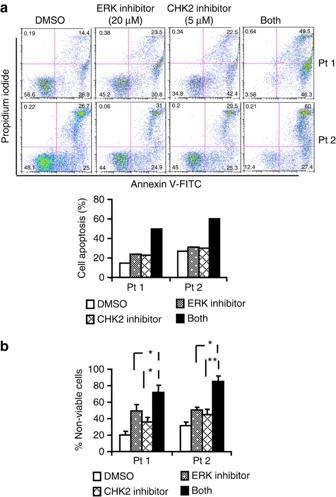Figure 7: ERK and CHK2 inhibitors enhance apoptosis induction in primary human DLBCL cells. (a) Single-cell suspensions were obtained from lymph node biopsies of patients diagnosed with DLBCL and were treated with DMSO, ERK inhibitor and CHK2 inhibitor II alone or in combination for 48 h after which the percentage of apoptotic cells was determined by Annexin V analysis as described in Methods. Flow cytometric profile was showed in the left panel. Pt 1, patient one; Pt 2, patient two. (b) Single-cell suspensions were treated as described in the (a). After the treatment, the percentages of non-viable cells were determined by trypan blue dye uptake in a hemocytometer. Data represents mean and s.d. from three separate experiments.Pvalues were calculated using a Studentt-test. *P<0.05; **P<0.01. Figure 7: ERK and CHK2 inhibitors enhance apoptosis induction in primary human DLBCL cells. ( a ) Single-cell suspensions were obtained from lymph node biopsies of patients diagnosed with DLBCL and were treated with DMSO, ERK inhibitor and CHK2 inhibitor II alone or in combination for 48 h after which the percentage of apoptotic cells was determined by Annexin V analysis as described in Methods. Flow cytometric profile was showed in the left panel. Pt 1, patient one; Pt 2, patient two. ( b ) Single-cell suspensions were treated as described in the ( a ). After the treatment, the percentages of non-viable cells were determined by trypan blue dye uptake in a hemocytometer. Data represents mean and s.d. from three separate experiments. P values were calculated using a Student t -test. * P <0.05; ** P <0.01. Full size image Our study addresses the therapeutic targeting and functional interaction between ERK and CHK2 in the setting of DLBCL. Our immunohistochemical analysis on tissue microarrays showed that both ERK and CHK2 protein levels were elevated in the majority of human DLBCL samples as compared with the normal GCB cells of reactive lymph nodes. This supports their value as potential therapeutic targets. The potential utility of ERK targeted therapy is supported by our previous data that treatment with the ERK inhibitor has marked antitumour activity in human DLBCL xenograft models [14] . Previous reports using western blotting have shown that CHK2 protein expression level is high in most primary diffuse large B-cell lymphomas (41/43), and absent or very low in six samples of normal peripheral blood lymphocytes [26] , which is consistent with our results. However, their western blot data also showed that CHK2 protein levels in DLBCL samples was similar to that in 6 reactive lymphoid tissues [26] . This discrepancy may be explained by the presence of other cell types such as T cells, follicular dendritic cells and stromal cells in addition to reactive B cells in the reactive germinal centre that was examined by western blot analysis. Furthermore, we were able to demonstrate using IHC that CHK2 levels of GC subtype of DLBCL are also elevated as compared with the normal GC cells. The mechanism for elevated CHK2 protein levels in DLBCL is still poorly described. Further experiments are necessary to investigate CHK2 modification and the CHK2 signalling network in DLBCL. It has been previously reported that Raf/MEK/ERK signalling was linked to DNA damage response and DNA repair through an ATM-dependent process [13] . This indicates that ERK is related with CHK2 signalling. We for the first time demonstrate the physical interaction between ERK1/2 and CHK2 and their co-localization in primary DLBCL cells. In addition, the interaction between CHK2 and ERK is disrupted by both CHK2 inhibitor II and CHK2 mutation at Thr68. We also found that ERK protein level is strongly correlated with the level of CHK2 protein (Pearson correlation coefficient ρ =0.737). These data together suggest that the interaction between ERK and CHK2 is likely to have biological relevance in DLBCL. This is further supported by our finding that inhibition of CHK2 phosphorylation of T68 disrupted the interaction between these two proteins. Thus, the functional interaction between ERK and CHK2 requires CHK2 phosphorylation. However, the ability for CHK2 to inhibit ERK phosphorylation of downstream substrates is kinase-independent and likely involves steric hindrance of ERK accessibility to substrate proteins. Determination of the molecular contacts involved in CHK2 interactions with ERK2 will provide insight into how CHK2 negatively regulates ERK functions. We found that inhibition of CHK2 activity modestly induced apoptosis of SUDHL4, SUDHL6 and Farage cells. CHK2 inhibition also induced DNA breaks by itself, manifested by increased phosphorylation of histone H2AX at serine 139. Inhibition of CHK2 expression has also been found to attenuate DNA damage-induced cell cycle checkpoints and to enhance apoptotic activity in HEK293 cells [19] . Targeting of CHK2 with siRNA enhanced apoptosis following induction of DNA damage by IR or doxorubicin, and inhibited the growth of resistant in vivo tumours [9] , [12] . Thus, induction of DNA damage by CHK2 inhibition may contribute to its antitumour activity. It should be noted that the response of a tumour to CHK2 manipulation depends on a specific cellular context. An intriguing proposal put forth by Laurent Antoni and his colleagues is that CHK2 kinase is similar to the two sides of the same coin [10] . In the case of wild-type CHK2 tumours that possess other defects in checkpoint and repair pathways, short-term inhibition of CHK2 could have therapeutic value [10] . In contrast, in those tumours where CHK2 function is diminished or eliminated, inhibition of other proteins involved in checkpoint and repair pathways might be lethal [10] . Defining how CHK2 kinase elicits such distinct cellular outcomes as cell survival through DNA repair versus apoptosis or senescence, depending on the genetic background is a critical area of investigation. The Ras/MEK/ERK signalling cascade is key pathway implicated in hematopoietic malignant cells survival signalling. Under physiologic conditions, ERK activation stimulates transcription leading to cell cycle progression and proliferation by activated growth factor signalling. ERK1/2 signalling has been implicated in attenuation of DNA damage through positive regulation of DNA repair mechanism [15] . Although the CHK2 inhibitor induced DNA breaks and damage, an unexpected finding was that inhibition of CHK2 activity leads to activation of ERK, which may preserve cell survival and proliferation. This provides a plausible explanation for the modest induction of cell apoptosis by CHK2 inhibitor and suggests that activation of ERK signalling pathway may represent a compensatory response to CHK2 inhibition. In other words, functional CHK2 may be required for cells to survive the basal level of genomic instability known to be present in many malignancies. However, the resulting ERK activation in response to CHK2 inhibition provides a potent survival signal that attenuates the apoptotic drive. This also provides a molecular mechanism by which interruption of ERK functions potentiates the killing of DLBCL cells treated with the CHK2 inhibitor. Similarly, the CHK1 inhibitor, UCN-01, also triggers compensatory activation of the prosurvival Ras/MEK/ERK cascade in various tumour cell types, including human multiple myeloma cells [15] . Our data is consistent with the previous report that activation of ATM by radiation downregulates phospho-ERK1/2 and its downstream signalling in both cell culture and tumour models [27] . It is imperative to identify drugs that can improve the efficacy and reduce the toxicity of standard anti-lymphoma therapy [28] . We have demonstrated that a novel ERK2 inhibitor enhances the antitumour activity of CHK2 inhibition in a human DLBCL xenograft model and primary DLBCL cells from human patients. It is also worth noting that there was no evidence of toxicity in animals treated with either ERK or CHK2 inhibitors alone or in combination. Additionally, exposure of normal human B cells and fibroblasts to both ERK and CHK2 inhibitors revealed little cytotoxicity. The lack of apparent toxicity to normal tissues makes targeting both ERK and CHK2 signalling an attractive clinical approach. Moreover, making this potential combination clinically appealing is the fact that CHK2 activation occurs after exposure to commonly used chemotherapeutic agents in DLBCL therapy as well as IR, suggesting that incorporating this dual inhibitor strategy could increase the therapeutic efficacy of standard regimens without increasing side effects. In summary, we have shown a positive correlation between ERK and CHK2 expression in human DLBCL. ERK physically interacts with CHK2 and inhibition of CHK2 activates ERK, which may serve as a compensatory response to enhance cell survival. Thus, combined inhibition of ERK and CHK2 exerts a potent anti-tumour effect in a human DLBCL xenograft model and primary DLBCL cells from human patients and may provide a therapeutic advantage. Whether these findings can be extended to other types of lymphoma is unknown at present and warrants further investigation. Our study demonstrates the mechanistic basis for the therapeutic targeting of DLBCLs with inhibition of both ERK and CHK2 and provides a rationale for using this combinatorial therapy. Cell culture and treatments DLBCL (SUDHL4, SUDHL6 and Farage) cells were grown in RPMI 1640 (Invitrogen) containing 10% fetal bovine serum and 1% Penicillin/Streptomycin. HeLa and HEK293 cells were grown in DMEM (Invitrogen) containing 10% fetal bovine serum. ERK inhibitor no. 76 (3-(2-aminoethyl)-5-((4-ethoxyphenyl) methylene)-2,4-thiazolidine- dione, HCl) was purchased from Calbiochem. CHK2 inhibitor II (2-(4-(4-chlorophenoxy) phenyl)-1H-benzimidazole-5-carboxamide hydrate) was from Sigma Aldrich. Myc (or Flag)-Wild-type CHK2 (WT), and Myc (or Flag) -T68A CHK2 constructs were gifts from Dr Sheau-Yann Shieh. GFP–WT CHK2, GFP–T68D CHK2, GST–WT CHK2 and GST–Kinase inactive CHK2(KD) constructs were kindly provided by Drs Bahassi and Stambrook. HeLa and HEK293 cell transfections were done with Lipofectamine 2000 (Invitrogen). Specific oligo siRNAs for CHK2, and the negative siRNA control were obtained from Santa Cruz. Transfection experiments were performed using Amaxa Nucleofector kit V (Amaxa), program A-020. Primary cells De-identified tissue samples were obtained from patients in accordance with the guidelines and approval of the University of Maryland Medical School Institutional Review Board and conform to the Declaration of Helsinki. Single-cell suspensions were obtained from lymph node biopsies by physical disruption of tissues (using scalpels and cell restrainers), followed by cell density ficoll-gradient separation. Cell number and viability were determined by trypan blue dye exclusion with at least 70–80% viable cells before treatment exposure. Primary cells were cultivated in medium containing 80% RPMI and 20% human serum supplemented with antibiotics, L -glutamine and HEPES for 48 hours +/− drug treatment. Cells were exposed to varying doses of the ERK and/or CHK2 inhibitors as indicated. Assessment of cell apoptosis and percentage non-viable cells Cells were seeded at equal density and then treated with the ERK and/or CHK2 inhibitors in complete RPMI 1640 medium. Forty-eight or seventy-two hours after drug treatment, cells were collected and apoptosis was analysed by flow cytometry using Annexin V staining kit (Southern Biotech). After designated treatments, cells were stained with Trypan Blue (Sigma-Aldrich). The numbers of non-viable cells were determined by counting the cells that showed trypan blue uptake using a hemocytometer. Statistical significance between experimental conditions was determined using the Student's t -test. Co-immunoprecipitation and immunoblotting After the treatment, the cells were lysed in the buffer (20 mM Tris–HCl pH 7.4, 150 mM NaCl, 1 mM EDTA, 1 mM EGTA, 1% Triton X-100, 1 mM Na 3 VO 4 , 1 mg ml −1 aprotinin, 1 mg ml −1 leupterin and 1mM PMSF). Insoluble material was removed by centrifugation, and antibodies were added to lysates for 1 h at 4 °C. Antibodies were collected with protein A or protein G-sepharose beads, and protein complexes were washed three times at 4 °C with the lysis buffer. Immunoblotting was performed using standard methods. Rabbit polyclonal anti–CHK2 (Santa Cruz), Anti-pCHK2, anti-pERK1/2, anti-ERK1/2 (Cell Signaling) and anti-PARP (Enzo) antibodies were used at 1:1,000, whereas anti-γH2AX (Millipore) and anti-actin (C2, Santa Cruz) were used at 1:5,000. Glutathione S -transferase fusion protein pull-down assays GST fusion proteins were expressed in Escherichia coli BL21(DE3) cells, and purified using glutathione-Sepharose beads. Briefly, the GST fusion proteins were coupled to glutathione beads at 4 °C for 1 h and then washed three times with the lysis buffer. The immobilized GST fusion proteins were incubated with the cell lysates for 1 h at 4 °C. The beads were washed with the lysis buffer four times and then the protein complexes were loaded in 10% SDS–PAGE, followed by immunoblotting. In vitro kinase assay ERK2 was expressed in bacteria and purified as previously described [29] . The GST-tagged Chk2 wild type and kinase inactive mutant (KD) was obtained from Drs Bahassi and Stambrook and expressed in bacteria [14] . ERK2 wild type (2 μg) and 0.5 μg MBP were incubated in the presence or absence of 1 μg GST–Chk2 wild type or inactive GST–Chk2 (KD) for 15 min at 300C in 50 mM Tris–HCl, 10 mM MgCl 2 , 1 mM EGTA, 2 mM DTT, 0.01% Brij 35 (pH 7.5) containing 20 μM cold ATP and 2 μCi γ- 32 P–ATP. Reactions were stopped with an equal volume of 2×SDS–PAGE sample buffer, and the proteins were resolved by SDS–PAGE, stained with Coomassie Blue, and phosphorylation of Chk2, ERK2 and MBP was determined by autoradiography or phosphoimager analysis. Tissue microarrays and protein detection Eight tissue microarrays were purchased from Biomax (#LM801). These arrays included a total of 10 reactive lymph nodes, 54 DLBCL and 6 other types of lymphoma. Four more DLBCL were excluded because of fall-off of the tissue sections during staining. Six of the 10 reactive lymph nodes were excluded in this analysis because of their lack of germinal centres. In addition, 20 reactive lymph node samples were provided by the UMGCC Pathology Biorepository and Research Core to serve as normal GCB controls. Human sample studies have been approved by the University of Maryland Medical School Institutional Review Board and conform to the Declaration of Helsinki. The paraffin sections were routinely stained with hematoxylin-eosin (H&E) reagents for morphologic examination. The Vectastain Elite ABC kit, purchased from Vector Laboratories, was used for immunohistochemical analysis.The paraffin sections were incubated overnight at 4 °C with the primary antibody. Anti-Ki67 and anti-CD20 antibodies (Dako) were used at 1:1,000. Anti-CD10,anti-BCL6 and anti-MUM1 antibodies (Abcam) were used at 1:20 and anti-FOXP1 antibody (Abcam) was used at 1:1,200. Anti-ERK1/2 antibody (Cell Signaling) was used at 1:300 and anti-CHK2 antibody (Santa Cruz) was used at 1:200. Slides were then treated with biotinylated secondary antibody and incubated with performed avidin–peroxidase complex. The sections were counterstained with hematoxylin, dehydrated, and mounted. Appropriate positive and negative controls were included in each assay. Immunohistochemical staining was evaluated independently by two hematopathologists (XFZ and SL with an inter-observer consistency >90%), according to our scaled criteria: 0, <25% neoplastic cells staining; 1+, 26–50% neoplastic cells staining; 2+, 50–75% neoplastic cells staining; 3+, >75% neoplastic cells staining. Based on the intensity of staining, the lymphomas were also divided into negative, weak, and strong staining patterns. Because the staining intensity may vary from assay to assay, our scaled criteria overrule the staining intensity, if only small number of lymphoma cells show strong staining. Occasional inter-observer inconsistencies were reconciled by re-reviewing together by the two hematopathologists to reach agreement. In combination, the lymphomas were roughly divided into negative (0 and/or negative), low (1+ and/or weak) and high (2+, 3+ and strong) expresser groups. The images were acquired with a Nikon eclipse 50i microscope (Nikon Instruments) and formatted with Adobe PhotoShop CS software. For fluorescence double staining, the section was treated as above and first stained with mouse monoclonal anti-ERK1/2 antibody (Cell Signaling, 1:300). After biotin blocking, the section was then stained with rabbit polyclonal anti-CHK2 antibody (Santa Cruz, 1:200). The sections were then washed with PBS and incubated with goat anti-rabbit Alexa Fluor 488 and goat anti-mouse Alexa Fluor 568 at a concentration of 1:200 each. The stained sections were mounted using Vectashield mounting medium (Vector). Control sections were similarly processed, except that the primary antisera were omitted, which yielded no staining. Images were captured using an Olympus FV1000 confocal microscope (Olympus) and processed with the Olympus Fluoview Version 1.7c software. In vivo tumour growth in the xenograft models All procedures involving animals were approved by the Institutional Animal Care and Use Committee of the University of Maryland. Female SCID Beige mice were housed in a pathogen-free environment under controlled conditions of light and humidity and received food and water ad libitum . SUDHL6 cells (1.2×10 6 ) were resuspended in 100 μl PBS and then mixed with an equal volume of Matrigel. The mixture was s.c. injected into the left and right dorsal flanks of 5- to 7-week-old female SCID mice. When the tumour reached the size of 60–163 mm 3 , the treatment was administered intraperitoneally every other day for a total of 20 days. ERK inhibitor no. 76 in DMSO was freshly prepared in PBS for a final dose of 5 mg kg −1 . CHK2 inhibitor II in alcohol was diluted in PBS for a final dose of 1 mg kg −1 . Injection of the vehicle alone was used as a control. Tumours were measured three times a week with calipers, and tumour volumes were calculated by the formula ½× r 1 2 × r 2 ( r 1 < r 2 ). At the moment of death, tumours were collected for further analysis. The significance of differences between treatment arms was determined using the Student's t -test. How to cite this article: Dai, B. et al . Functional and molecular interactions between ERK and CHK2 in diffuse large B-cell lymphoma. Nat. Commun. 2:402 doi: 10.1038/ncomms1404 (2011).